Craniometric analysis of European Upper Palaeolithic and Mesolithic samples supports discontinuity at the Last Glacial Maximum The Last Glacial Maximum (LGM) represents the most significant climatic event since the emergence of anatomically modern humans (AMH). In Europe, the LGM may have played a role in changing morphological features as a result of adaptive and stochastic processes. We use craniometric data to examine morphological diversity in pre- and post-LGM specimens. Craniometric variation is assessed across four periods—pre-LGM, late glacial, Early Holocene and Middle Holocene—using a large, well-dated, data set. Our results show significant differences across the four periods, using a MANOVA on size-adjusted cranial measurements. A discriminant function analysis shows separation between pre-LGM and later groups. Analyses repeated on a subsample, controlled for time and location, yield similar results. The results are largely influenced by facial measurements and are most consistent with neutral demographic processes. These findings suggest that the LGM had a major impact on AMH populations in Europe prior to the Neolithic. The Last Glacial Maximum (LGM) represents the most severe climatic event since anatomically modern humans (AMH) arrived in Europe ~45 ka BP [1] . Beginning as early as 26.5 ka BP, with amelioration beginning after 20 ka BP [2] , it resulted in the extension of land-based ice sheets over much of the continent, with a lowering of sea level by ~130 m [3] , and a reduction in air surface temperatures by 8–15 °C below present-day values [4] . The major climatic and environmental changes that preceded the LGM led to a contraction in the range of European human populations. The progressive depopulation of much of the continent by humans north of the Mediterranean basin resulted in the formation of regional refugia after 25 ka BP [5] . In contrast to the ‘open systems’ [6] that have been hypothesized for pre-LGM populations, gene flow would have become more localized within refugia. It is speculated that populations occupying more northern latitudes migrated into refugial zones, while others may have gone extinct [5] . Genetic and phenotypic variation would likely have been affected by drift and founder events as populations became more fragmented [7] . This may have created a population bottleneck, which could conceivably have resulted in significant phenotypic changes in post-LGM groups due to drift. It is likely that many populations remained in isolation until after the LGM, after which time groups moved out from refugia to occupy regions that had been left uninhabited. There is evidence to suggest significant biological differences between pre- and post-LGM groups. It has been long recognized that pre-LGM people were taller than in succeeding periods [8] . Meiklejohn and Babb [9] noted a sharp decrease in long-bone length between pre- and post-LGM populations, with no further changes through the Holocene. Similar conclusions were reached by Formicola and Holt [10] , who singled out the LGM as ‘a watershed in body size of these populations’. The decrease in lower limb lengths coincides with a reduction in lower limb robusticity between pre-LGM and late glacial groups [11] , contrasting with an increase in upper limb muscularity and robusticity [12] . The post-LGM postcranium has been interpreted within an adaptive framework as selection acting over the long term to produce a more cold-adapted body size and shape [13] . Since postcranial dimensions are affected considerably by environmental factors [14] , they can be an unreliable proxy for reconstructing population history. As a result, it is hard to determine to what degree disparities between pre-LGM and later groups reflect population history. Changes in the postcrania may simply reflect an adaptive response to environmental stress associated with the LGM. In contrast, craniometric studies demonstrate that overall cranial shape variation in modern humans results in large part from neutral evolutionary forces [15] , [16] ; a correspondence that makes cranial data a useful genetic proxy for reconstructing population histories. A key issue in this regard is the extent of changes, if any, within pre-LGM cranial morphology. There has been a tendency to see modern European cranial characteristics as largely established by the pre-LGM, with little or no change thereafter [17] . The study of morphometric variation after this period was seen as contributing little to major questions in human evolution—a view that derived validation from work by Morant [18] , who saw pre-LGM and late glacial cranial morphology as largely modern, and strikingly homogeneous in space and time. Subsequent changes were often viewed as being cultural rather than biological [17] , [19] . Hence, this represents the first assessment of the effects of the LGM on patterns of craniometric variation in European Late Pleistocene and Holocene humans. Given the geographically and temporally disparate nature of the data set, we were unable to construct population units, demes or operational taxonomic units as have been used in previous studies of prehistoric European cranial series [20] . This precluded the detailed testing of alternative evolutionary models of population dispersal, isolation or climatic selection. However, the basic hypothesis that the LGM represents a major chronological marker in terms of overall morphological continuity across Europe could be adequately tested using our data. In addition, the likely effects of three major confounding factors were assessed via a series of post hoc analyses. First, systematic differences in absolute cranial size across chronological groups could bias the analyses in favour of finding significant differences between groups, especially if allometric patterns change through time. Accounting for potential differences in scaling is also important given the uncertainties surrounding the sex ratios of each sample. Hence, controlling for isometric scaling differences among groups also allowed differing patterns of sexual size dimorphism to be constrained. Second, given the uneven geographic distribution of specimens within each of the four major chronological groups, any systematic differences between groups could be due to spatially mediated factors. Therefore, we performed a post hoc analysis focusing on three core regions (Central Europe, Italy and southern France) for which data were available for pre- and post-LGM samples. Finally, given that our pre- and post-LGM groups are necessarily chronologically arranged, any systematic differences found might be attributable to the effects of morphological divergence simply as a result of time. Hence, we performed an additional post hoc analysis to illustrate that temporal distance alone does not explain the divergence patterns observed among the pre- and post-LGM specimens. The results of a multivariate analysis of variance (MANOVA) on size-adjusted cranial measurements show significant differences across the four periods. A discriminant function analysis shows separation between pre-LGM and later groups. Analyses repeated on a subsample controlled for time and location gives similar results. The results are largely influenced by facial measurements and are most consistent with neutral demographic processes. Furthermore, the results are not consistent with an accelerated rate of evolution during the post-LGM. These findings suggest that the LGM had a major impact on AMH populations in Europe prior to the Neolithic. Complete data set A MANOVA of all four chronological groups found them to be significantly different using Pillai’s trace ( V (30, 558)=0.571, P <0.001). The assumption that the covariance matrices are the same across the groups could not be rejected at the recommended α -value of 0.001 (Box’s χ 2 =165, P =0.027; Box’s F (165, 17527.3)=1.21, P =0.036). 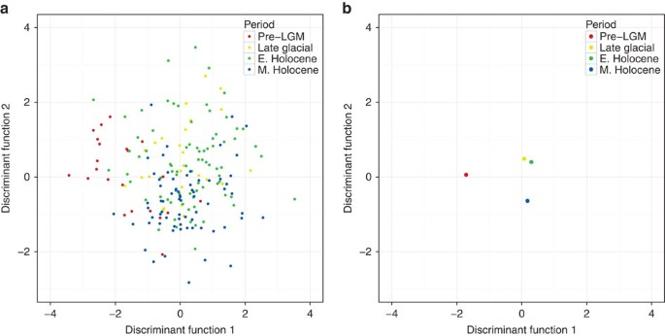Figure 1: Discriminant function plots for complete data set. (a) Score plot of the first two discriminant functions on size-adjusted craniometric measurements. Each circle represents an individual from one of the four groups: Pre-LGM (red), late glacial (yellow), Early Holocene (green) and Middle Holocene (blue). (b) Mean of each group in the score plot. The linear discriminant function analysis revealed three discriminant functions ( Table 1 ). The first function explained 52% of the variance, while the other two explained 34% and 14%, respectively. A plot of the first two discriminant functions, along with a separate plot of their mean scores ( Fig. 1 ), show that the pre-LGM is discriminated from the other groups along the first discriminant function. The late glacial and Early Holocene groups cluster together. The coefficients of the discriminant functions revealed that the first function differentiated nasal height, nasal width, orbital height and least frontal breadth. Box plots of these particular measurements are shown in Fig. 2 . The pattern suggests that the pre-LGM group had relatively greater values for nasal dimensions. The second discriminant function differentiated facial dimensions, specifically nasal height, nasal width, orbital height and orbital breadth. Cross-validation ( Supplementary Table 1 ) shows that the model performs well above what would be expected by chance (25% for each group), except in the case of the late glacial group, which was misclassified as Early or Middle Holocene 76% of the time. Table 1 Function loadings of discriminant function analysis for size-adjusted craniometric data. Full size table Figure 1: Discriminant function plots for complete data set. ( a ) Score plot of the first two discriminant functions on size-adjusted craniometric measurements. Each circle represents an individual from one of the four groups: Pre-LGM (red), late glacial (yellow), Early Holocene (green) and Middle Holocene (blue). ( b ) Mean of each group in the score plot. 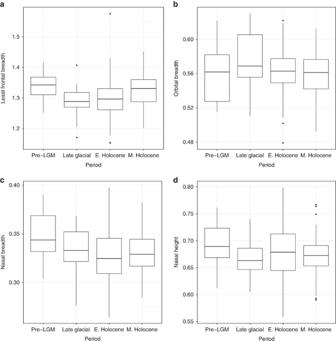Figure 2: Box plots of size-adjusted craniometric measurements with the highest loadings for the first discriminant function. (a) Least frontal breadth, (b) orbital breadth, (c) nasal breadth and (d) nasal height. The line inside the box marks the median. The upper and lower hinges correspond to the 25th and 75th percentiles. The upper and lower whiskers extend to the highest and lowest values that are within 1.5 times interquartile range of the hinge. Outlying data beyond this are plotted as points. Pre-LGM (n=22), late glacial (n=25), Early Holocene (n=79) and Middle Holocene (n=71) groups. Full size image Figure 2: Box plots of size-adjusted craniometric measurements with the highest loadings for the first discriminant function. ( a ) Least frontal breadth, ( b ) orbital breadth, ( c ) nasal breadth and ( d ) nasal height. The line inside the box marks the median. The upper and lower hinges correspond to the 25th and 75th percentiles. The upper and lower whiskers extend to the highest and lowest values that are within 1.5 times interquartile range of the hinge. Outlying data beyond this are plotted as points. Pre-LGM ( n =22), late glacial ( n =25), Early Holocene ( n =79) and Middle Holocene ( n =71) groups. Full size image Next, we calculated the squared Mahalanobis distances between group means. These are presented in Table 2 , with associated F - and P -values. The distances between the pre-LGM and all other groups were between twice and four times greater than any of the distances among the post-LGM groups. Table 2 The squared Mahalanobis distance between group means. Full size table The hypothesis of equality of variances of the geometric means (an indirect measure of absolute cranial size) across the four temporal groups was rejected using Levene’s test, F (3, 193)=3.990, P =0.010. Welch’s test was used, since the homogeneity of variance assumption is required by ANOVA. Absolute cranial size did not differ significantly among the four temporal groups, Welch’s F (3, 65.304)=1.473, P =0.230. This indicates that scaling differences cannot explain any systematic among-group divergence patterns. The two-tailed Mantel test of temporal distance and morphological distance was also not statistically significant ( r =0.001; P =0.836) demonstrating that temporal distances among specimens do not predict their morphological distances. Therefore, despite the fact that the four groups tested are chronologically defined, any systematic among-group differences cannot be attributed to temporal distance alone. Nasal indices (nasal breadth relative to nasal height), were not found to differ significantly among the four chronological groups (Welch’s F (3, 63.395)=1.480, P =0.183). Subsample constrained by geography A MANOVA of the three chronological groups (pre-LGM, late glacial and Early Holocene) constrained by three core geographic regions (Central Europe, Italy and southern France) found them to be significantly different using Pillai’s trace ( V (20, 128)=0.656; P <0.001). A Box’s M -test for the homogeneity of covariance matrices across the three groups was not significant at an α -value of 0.001 (Box’s χ 2 =138, P =0.036; Box’s F (110, 10,466)=1.24, P =0.047). 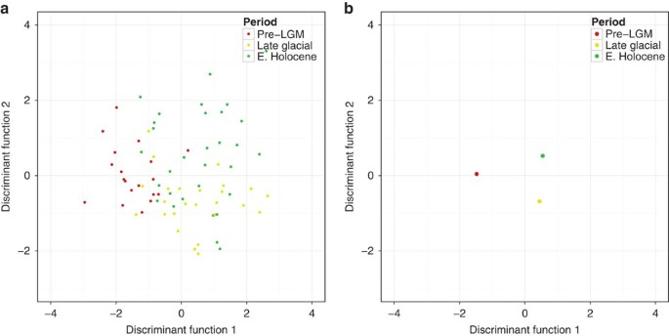Figure 3: Discriminant function plots for subsample constrained by geography. (a) Score plot of the first two discriminant functions on size-adjusted craniometric measurements in subsample constrained by geography. Each circle represents an individual from one of the three groups: pre-LGM (red), late glacial (yellow) and Early Holocene (green). (b) Mean of each group in the score plot in subsample constrained by geography. The linear discriminant function analysis revealed two discriminant functions ( Table 3 ). The first function explained 73.3% of the variance, while the second explained 26.7%. A plot of the first two discriminant functions, along with a separate plot of their mean scores ( Fig. 3 ), show that the pre-LGM is discriminated from the other two groups along the first discriminant function. The coefficients of the discriminant functions revealed that the first function differentiated orbital height, nasal breadth, orbital breadth and nasoalveolar height. Box plots of these particular measurements are shown in Fig. 4 . The pre-LGM group had relatively smaller values for orbital measurements and nasoalveolar height, and greater values for nasal breath. The second discriminant function differentiated facial dimensions, specifically nasal height, nasal breadth, orbital height and orbital breadth. Cross-validation ( Supplementary Table 2 ) shows that the model performs well above what would be expected by chance (25% for each group). Table 3 Function loadings of discriminant function analysis for size-adjusted craniometric subsample constrained by geography. Full size table Figure 3: Discriminant function plots for subsample constrained by geography. ( a ) Score plot of the first two discriminant functions on size-adjusted craniometric measurements in subsample constrained by geography. Each circle represents an individual from one of the three groups: pre-LGM (red), late glacial (yellow) and Early Holocene (green). ( b ) Mean of each group in the score plot in subsample constrained by geography. 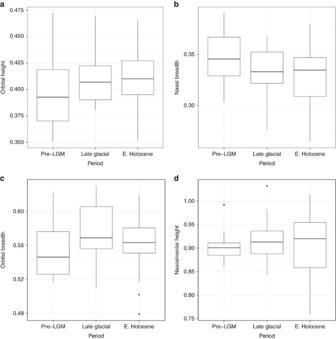Figure 4: Box plots of size-adjusted craniometric measurements with the highest loadings for the first discriminant function in subsample constrained by geography. (a) Orbital height, (b) nasal breadth, (c) orbital breadth and (d) nasoalveolar height. The line inside the box marks the median. The upper and lower hinges correspond to the 25th and 75th percentiles. The upper and lower whiskers extend to the highest and lowest values that are within 1.5 times interquartile range of the hinge. Outlying data beyond this are plotted as points. Pre-LGM (n=19), late glacial (n=25) and Early Holocene (n=31) groups. Full size image Figure 4: Box plots of size-adjusted craniometric measurements with the highest loadings for the first discriminant function in subsample constrained by geography. ( a ) Orbital height, ( b ) nasal breadth, ( c ) orbital breadth and ( d ) nasoalveolar height. The line inside the box marks the median. The upper and lower hinges correspond to the 25th and 75th percentiles. The upper and lower whiskers extend to the highest and lowest values that are within 1.5 times interquartile range of the hinge. Outlying data beyond this are plotted as points. Pre-LGM ( n =19), late glacial ( n =25) and Early Holocene ( n =31) groups. Full size image Following the discriminant function analysis, the squared Mahalanobis distances between group means were calculated. These are presented in Table 4 alongside associated F - and P -values. The distances between the pre-LGM and all other groups were approximately three times larger than the distances among the two post-LGM groups. In addition, the pre-LGM group was significantly different from the two post-LGM groups, while the post-LGM groups were statistically indistinguishable from each other. Table 4 The squared Mahalanobis distance between group means of subsample constrained by geography. Full size table This study used craniometric data to explore temporal and geographic variation in pre- and post-LGM specimens, using a large, well-dated data set for these periods. The pre-LGM showed greatest divergence in our analyses, pointing to the LGM as a disruptive event in the population history of Europe. No clear morphological division was detected between the late glacial and Holocene groups, suggesting that the division between them is arbitrary from a biological perspective. Multivariate statistical analyses found significant differences across the four time periods, with the greatest divergence occurring between the pre-LGM group and combined post-LGM groups. In a linear discriminant analysis, the first discriminant function differentiated between the pre-LGM and all other groups. The Mahalanobis squared distances between the group means were larger for comparisons with the pre-LGM group. The misclassification of the late glacial group as Holocene suggests that they share greater affinities with Holocene rather than pre-LGM specimens. This is further suggested by the small Mahalanobis distance between the late glacial and Early Holocene groups along the first two discriminant axes. These findings are supported further by the results showing that temporal distance alone cannot explain inter-specimen morphological divergence and that no systematic scaling differences could be observed among the four groups. In addition, the analyses focusing on three core geographic areas found that the pre-LGM specimens from these regions were statistically different from post-LGM specimens from the same regions, while post-LGM groups were statistically indistinguishable from one another. While there are detectable craniometric differences between the pre-LGM and later groups, it is not clear to what extent these result from neutral evolutionary forces or natural selection. The largest loadings for the discriminant function analysis were on middle and upper facial measurements, specifically orbital and nasal dimensions, least frontal breadth and nasoalveolar height. Previous studies on modern crania reported facial shape to be a relatively poor indicator of past population history [15] , [21] . Aspects of facial shape variation have also been linked to climate [15] , [22] , [23] . The observation that post-LGM groups tend to have smaller nasal dimensions could be consistent with the expected adaptive response to cold climate [24] . However, nasal indices, which are generally found to differ between cold- and warm-adapted human populations [22] , were not found to differ significantly among the four chronological groups, suggesting that thermoregulatory adaptation is not responsible for these morphological patterns. One possible explanation may lie in the correlation between nasal dimensions and overall body size, which has been suggested [25] to reflect the increased metabolic and oxygen consumption needs of overall larger bodies. Therefore, if the post-LGM populations of Europe also underwent a significant decrease in overall body size, as has been suggested based on analyses of postcranial material [9] , [10] , it would explain why relative nasal dimensions also decreased in specimens of the late glacial and Early Holocene periods. Previous analyses of globally distributed populations have suggested that absolute differences in cranial size may be consistent with climatically driven adaptation according to Bergman’s rule [26] . Our findings regarding the nasal index, and the fact that cranial size did not vary systematically among the pre- and post-LGM groups, point to non-climatically mediated divergence based on alternative stochastic evolutionary factors. While we cannot rule out the possibility of climatically driven adaptation across the LGM, our results are more consistent with other (neutral) demographic population processes, such as population isolation, migration and genetic drift causing the divergent patterns we see between pre- and post-LGM populations. Another possibility is that the statistical divergence we see between pre- and post-LGM groups is due to differing rates of evolution across the LGM. We assessed this by calculating Darwin units using the discriminant function scores. Results show no consistent pattern and suggest that there was no substantial change in the per-generation rate of evolution across the LGM. The archaeological hiatus for much of Northern and Central Europe during the LGM suggests that people abandoned these regions, with a few isolated exceptions [27] . The size of populations surviving in refugial zones is unclear, although it is thought that these increased in size due to an influx of migrants from further north. This view derives support from the archaeological record, which documents a marked increase in the number of sites in southern France [28] and Iberia [29] . It may also be assumed that there were sufficiently large refugial populations to fuel post-LGM expansion into Northern Europe [30] . Around the time of the LGM, refugial populations in Southern Europe would have been isolated from one another, allowing for the divergence in the expression of phenotypic traits. For instance, Italy was cut off from refugia in Western Europe by the glaciated Alps, while to the east the Western Balkans seem to have been only sparsely populated [31] . As temperatures began to rise during the Bølling interstadial, late glacial groups repopulated the continent. The low resolution of data makes it difficult to comment on whether craniometric changes were due to differences in the population structure between refugial groups during the LGM or resulted from population bottlenecks during founder events associated with the recolonization of the continent. Our findings are congruent with genetic studies that indicate that only a small fraction of modern European mitochondrial DNA (mtDNA) is derived from the pre-LGM; the vast majority coming from the late glacial expansion from Southern European and Near Eastern refugia [32] , [33] . MtDNA studies point to a number of haplogroups that likely arose in the Franco-Cantabrian refugium [34] , [35] . Evidence for new haplogroups originating in the Balkans [36] and Ukraine [37] add weight to claims that they were also important LGM refugia [38] . A recent study of mtDNA markers of Upper Palaeolithic and Mesolithic populations suggests some genetic continuity between pre- and post-LGM European hunter-gatherers [39] . The great majority of pre-agricultural groups belong to the haplogroup U, within which subhaplogroup U5 was the most ancient. Its date, based on calibration of the mitochondrial clock, is ~30 ka. The absence of evidence for continuity in other subhaplogroups, however, may point to changes in genetic structure brought about by an LGM bottleneck. In any case, mtDNA haplogroups cannot provide a comprehensive overview of the population history of these populations, which requires analysis of autosomal multilocus genomic data [40] . The pan-European approach adopted here and the small sample of available crania from the pre-LGM limits the ability to detect regional patterns of craniometric variation. Although not necessarily reflective of population events, archaeological evidence for continuity across the LGM varies between regions of the continent, as does the sequence of documented technocomplexes. In Cantabria, a number of sites with long stratigraphic sequences indicate continuity between the Solutrean and Magdalenian [41] . Some scholars recognize a sharp break between the Solutrean and Badegoulian [42] ; however, the nature of the latter is complex and may represent an eastern influence [43] . In contrast, in Central and Eastern Europe, and in the Italian and Balkan peninsulas, there is continuity of backed blade and bladelet technologies from the Gravettian into the so-called Epigravettian [31] , the latter being synchronous with the Solutrean through Azilian of Western Europe. Caramelli et al . [44] found that pre-LGM skeletal remains in Italy (Paglicci 23) had an mtDNA sequence still common in Europe, which may suggest continuity on the peninsula. Further evidence of continuity in Italy may be present in mortuary practices, with apparent continuity from the Gravettian into the Epigravettian [45] . On the basis of craniometry, this study suggests that European Upper Palaeolithic populations can be morphologically separated into two chronogroups (pre-LGM and late glacial), separated by the LGM. In addition, there is morphological continuity between late glacial and Holocene populations, a view supported by the archaeological record, which shows that many aspects of the Mesolithic extend back to the LGM [46] . The archaeological boundary reflects a cultural response to post-glacial conditions. The Mesolithic has been, and will likely remain, a difficult period to define. Attempts to find ‘distinctively Mesolithic’ features have repeatedly failed [47] . While microliths are ubiquitous during the Mesolithic, they are nonetheless present (albeit in smaller frequencies) during the Upper Palaeolithic [48] . Similarly, polished tools and ceramics, which had been thought to be characteristic of the Neolithic, are now known to occur in a number of later Mesolithic contexts [49] . Not surprisingly, our study finds that the division of the Mesolithic into early and late phases is similarly arbitrary in morphological terms. Data set The craniometric data set (see Supplementary Data 1 ) used here was developed by two of us (C.M. and R.P. ), with the assistance of Winfried Henke (Universität Mainz). Other Upper Palaeolithic and Mesolithic data sets have generally been less rigorous in their sample selection, often accepting earlier attribution of specimens without question. Three main issues were taken into consideration while compiling the data set: (1) the primary and secondary sources of measurements, (2) measurement protocols and (3) the archaeological ascription of sites and their specimens. Our aim was to maximize the number of individuals used, while applying rigorous control over the included specimens. Wherever possible, we used published and unpublished data collected by C.M. and R.P. However, in cases where we did not have access to material, we have collected published data. Furthermore, in many instances data from more than one source exists. For this reason, C.M. created a database providing separate entries for each data source (for example, Oberkassel 1 has 14 entries). This permitted us to identify any incongruities owing to mistakes in the original recording. Since some sources included measurements not recorded elsewhere, it also allowed us to maximize the number of possible observations for any given specimen in the final data set. A second issue concerned the measurement protocol used. There has been some change over the years in craniometric protocols. Ideally, we would have adopted the most recently developed measurement protocols (for example, those used in the description of the pre-LGM material from Mladeč [50] , [51] ); however, very few other series have been measured using these methods. In addition, lost or destroyed specimens (for example, the pre-LGM material from Dolní Věstonice, Mladeč and Předmostí were lost in the Mikulov fire in 1945) cannot be restudied using this procedure. For this reason we have used more traditional measurement methods. We collected these from three widely employed systems—Howells [52] , Martin and Saller [53] and the British Biometric System [54] —and a fourth developed by David Frayer (personal communication, system not published), which was used in the Mladeč studies cited above. Attention was paid to system equivalence (or lack thereof), since it is important that measurements reported under a general term are equivalent (for example, orbital breadth and auricular breadth are measured differently in different systems). The third issue concerned the correct archaeological ascription of specimens and sites. While a more rigorous approach has been employed for the Mesolithic [55] , [56] , surveys of the Upper Palaeolithic have been generally less critical and complete [57] . Basic information on within-site provenance of material is an issue. In the past decade, many finds, once thought to be secure on archaeological and/or stratigraphical grounds, were found to differ widely from their assumed age. Trinkaus’ [58] list of assumed pre-LGM specimens, now shown to be Holocene in age (most are post-Mesolithic), is particularly sobering. Although earlier, a list of presumed early Aurignacian fossils by Churchill and Smith [59] records several now directly dated to the Holocene. Finally, we have applied the protocol developed for a similar purpose, albeit on a different data set, by Pinhasi and Meiklejohn [9] , [60] . A critical criterion was that skeletal elements, or material from the immediate burial environment, were directly dated by 14 C methods. If dates were absent, then clear evidence for association of material and attributed cultural level was required (for example, the association of the Chancelade skeleton with the French Magdalenian). The sample was subdivided into four temporal groups—Pre-LGM, late glacial, Early Holocene and Middle Holocene—whose boundaries are defined primarily by major climatic events and secondarily by archaeological events. These periods are largely contemporaneous with the following cultural periods: the early Upper Palaeolithic, late Upper Palaeolithic, early Mesolithic and late Mesolithic. Skeletal remains were attributed to each of these periods based primarily on dating and secondarily on archaeological associations. Geoarchaeological framework The data set discussed above covers ~30 ka and two broad archaeological periods: the Upper Palaeolithic and Mesolithic. Geologically, this incorporates roughly the second half of the Würm/Weichsel glacial cycle and first half of the Holocene. Our cranial data set contains samples covering a large proportion of the four chronological periods defined above, and range in age from ~5 to 31 ka BP. They have been assigned to one of the four defined periods based primarily on dating and secondarily on archaeological associations. While the defined groups cannot be assumed to be bounded cultural or biological units, in the context of the hypothesis being tested, the use of these four chronologically defined groupings is appropriate. The first period, the pre-LGM, covers late marine isotope stage (MIS) 3 after ~35 ka BP. The early parts of this transition are marked by climatic oscillations, warmer (Greenland) interstadials and colder Heinrich events. After ~27.5 ka BP this phase is replaced by early MIS 2 (ref. 61 ) and extends to the LGM, which lasted at least six millennia in some regions [2] and ends in most places around 20 ka BP (24 ka cal BP). Archaeologically, the early Upper Palaeolithic (pre-LGM) begins with the appearance of the Aurignacian, which is generally attributed to AMH [62] . By ~30 ka, this is replaced by the Gravettian, especially noted for bone, ivory and antler implements, together with complex art and rich burials, lasting until ~20 ka BP and referred to as a ‘Golden Age’ [63] . Much of our pre-LGM sample derives from the Gravettian period. Archaeologically, the LGM covers the late Gravettian and the appearance of the Solutrean, as well as the more poorly understood Badegoulian. Compared with the Gravettian, which is found throughout much of the continent, the Solutrean is largely restricted to Western and Southwestern Europe—the Loire Valley is its approximate northern boundary. North and east of this an archaeological hiatus extends from southern Britain to Poland from the LGM to ~14 ka BP [64] . In Cantabria, there was a ‘boom’ in the number of Solutrean sites [65] . The apparent break in lithic technology seems to reflect a focus on projectile types designed to maximize hunting success under conditions of competition. Other technological innovations, such as the spear-thrower and eyed bone needle, are linked to hunting efficiency and the sewing of hide-based clothes. The second period, the late glacial, is associated with climatic amelioration during later MIS 2 and the slow retreat of continental ice sheets in Europe. It is associated with a rapid demic expansion out of glacial refugia, identified archaeologically as the Magdalenian, which continued through the set of cold/warm cycles during the terminal Pleistocene [5] . The Magdalenian appears to have developed in France earlier than in Iberia [65] , and marked a further change in technological investment, which saw the gradual replacement of classic points with ‘the compound weapon tip formed by resilient, reuseable antler points and low-investment, replaceable backed bladelets’ [29] . Straus [65] viewed this archaeological shift in the Iberian context within a continuity framework. There is also a shift in burial rituals, with the rich burials of the Gravettian being replaced by simpler inhumations. These are often single burials with fewer grave goods, although there are exceptions (for example, St-Germaine-la-Rivière). The Magdalenian later expands across much of Western and Central Europe. The third period, the Early Holocene, comprises the Preboreal and Boreal climatic phases. Following the late glacial climatic oscillations, the Holocene is marked by a rapid increase in temperature to near modern levels and rapid deglaciation. Archaeologically, this period is largely coeval with the early Mesolithic. The fourth and final period, the Middle Holocene, corresponds to the Atlantic climatic phase. For this study, the Early–Middle Holocene boundary was determined to be 7.4 ka BP, corresponding to the 8.2 ka cal BP cold event [66] . The end of this period is marked not by a climatic boundary but by the appearance of food production and the Neolithic. This period corresponds in most part with the late Mesolithic. We are agnostic on the dynamic of this final shift, which lies beyond the compass of this paper. Archaeologically, these Holocene periods are associated with the transition from the late Upper Palaeolithic to the Mesolithic and can be viewed as reflecting post-glacial adaptation. We concur with Price’s [47] view that the ‘Mesolithic means simply early late glacial hunter-gatherers, nothing more’. Certain regions saw more intensive settlements at this time, as overall population size increased [28] . Statistical analyses The analysed data consist of 197 crania (summary information is provided in Table 5 ; see Supplementary Data 2 for more detailed information on the specimens used). They were selected from the larger data set, discussed above ( Supplementary Data 1 ). Sample sizes for each of the four groups were 22 pre-LGM, 25 late glacial, 79 Early Holocene and 71 Middle Holocene specimens. Only adult specimens with radiocarbon dates or those with secure provenance were used in the analyses. A standard set of 10 Martin and Saller [53] craniometric measurements were used ( Supplementary Table 3 ), corresponding to essential height, width and length dimensions of the cranial vault and face (including orbital and nasal regions; eight are also defined in the same way by Howells [52] ). Specimens missing three (30%) or more measurements were dropped. Missing values were replaced by multiple regression estimates based on the entire data set (7% of measurements were estimated for the data set). Cranial measurements were transformed to size-adjusted shape variables via division by the geometric mean. Table 5 Sample summary. Full size table A MANOVA was carried out to assess whether cranial measurements were statistically significant across time periods. Unequal group sizes can cause the assumption of homogeneity of covariance matrices to be violated. This assumption was tested using Box’s M -test. This test is sensitive to violations of normality and an α -value of 0.001 is recommended [67] . A discriminant function analysis was performed in order to assess the magnitude of cranial shape disparity between the four temporal groups. Discriminant analysis determines a linear combination of the original variables, known as canonical discriminant function coefficients, which maximizes the separation between the groups defined a priori . Although the discriminant function analysis will attempt to maximize the differences between the groups we have defined a priori , it should be biased towards discriminating between all groups in a similar manner. Hence, if the LGM does not represent a major source of discontinuity, we should expect all four groups to be approximately equally different from each other. The adequacy of classification was assessed by cross-validation. Mahalanobis squared distances were calculated to determine the strength of the canonical variates in discriminating between group means. This dissimilarity measure rescales all variables to have equal variance, and takes into account the intercorrelations between the variables. The Mahalanobis distance is helpful in assessing which groups are most different. Prior probabilities were calculated in order to control for unequal sized groups. All data preparation and discriminant function analyses were carried out in R 3.0.2 (ref. 68 ). Box’s M -test and Mahalanobis squared distances between group means were calculated using Stata 12.1 (ref. 69 ). In many cases, the availability of multiple sources of data for individual specimens allowed us to identify and remove conspicuous errors. It was not possible, however, to assess the degree of interobserver error in the sample, although this factor should be kept in mind when interpreting the results. Thereafter, a series of three post hoc analyses were performed. First, to account for the possibility that absolute differences in cranial size might be influencing the results, we applied Welch’s test (an alternative to ANOVA in cases where assumption of homogeneity of variances has been violated) to the geometric mean data across all four groups. Second, we tested for the congruence between temporal distance and morphological distance to assess whether the passage of time alone might explain any systematic differences observed among the four temporal groups. A Euclidean distance matrix was generated from the 10 cranial shape variables for all 197 specimens and this was statistically compared against an equivalent matrix based on temporal distance using a two-tailed Mantel test. In cases where absolute 14 C dates were not available for particular specimens, the average age for that temporal group was used instead (see Table 5 ). The third post hoc test assessed the likely effect of geographic distribution of specimens on the initial results obtained. All specimens were divided into one of nine geographic regions (see Supplementary Data 1 ). Of these nine regions, only two (Central Europe and southern France) were represented across all four temporal groups, and in the case of the Middle Holocene group, only three specimens from Central Europe were available. Given that using only these two core regions results in very small sample sizes, it was decided to focus on three core regions (Central Europe, Italy and southern France) for the pre-LGM ( n =19), late glacial ( n =25) and Early Holocene ( n =31) groups. The same statistical procedures were applied as before (MANOVA, discriminant function analysis and Mahalanobis distances) in order to check if geographic distribution might affect the initial results obtained. Rate of evolution We explored the possibility that the results could be explained by a faster per-generation rate of evolution in the three post-LGM groups. Darwin units were calculated using the first three discriminant functions and these were plotted versus the number of generations (one human generation=29 years) that passes based on absolute time intervals calculated from the median dates for each pairwise group. A Darwin unit is defined as one logarithmic increase in the phenotypic value of a trait for each million year of evolution [70] and is described by the equation where X 1 and X 2 are the mean trait values and Δ t is the change in time in millions of years. The observed rate of evolution ( Supplementary Figs 1–3 ) is not consistent with the hypothesis that the rate of evolution accelerated during the post-LGM. How to cite this article: Brewster, C. et al . Craniometric analysis of European Upper Palaeolithic and Mesolithic samples supports discontinuity at the Last Glacial Maximum. Nat. Commun. 5:4094 doi: 10.1038/ncomms5094 (2014).